Loss of neuronal 3D chromatin organization causes transcriptional and behavioural deficits related to serotonergic dysfunction The interior of the neuronal cell nucleus is a highly organized three-dimensional (3D) structure where regions of the genome that are linearly millions of bases apart establish sub-structures with specialized functions. To investigate neuronal chromatin organization and dynamics in vivo , we generated bitransgenic mice expressing GFP-tagged histone H2B in principal neurons of the forebrain. Surprisingly, the expression of this chimeric histone in mature neurons caused chromocenter declustering and disrupted the association of heterochromatin with the nuclear lamina. The loss of these structures did not affect neuronal viability but was associated with specific transcriptional and behavioural deficits related to serotonergic dysfunction. Overall, our results demonstrate that the 3D organization of chromatin within neuronal cells provides an additional level of epigenetic regulation of gene expression that critically impacts neuronal function. This in turn suggests that some loci associated with neuropsychiatric disorders may be particularly sensitive to changes in chromatin architecture. Research over the last decade indicates that epigenetic dysregulation importantly contributes to the aetiology of neuropsychiatric disorders [1] , [2] , [3] . Among the different epigenetic mechanisms of regulation of gene expression, the modulation of higher-order chromatin structures is one of the least understood. The interior of the eukaryotic cell nucleus is a highly organized 3D structure in which regions of the genome that are millions of bases apart, even belonging to different chromosomes, work together and define specialized sub-structures with dedicated functions [4] , [5] . Thus, in most interphase somatic cells, pericentromeric regions are organized in clusters referred to as chromocenters that consist of transcriptionally silent DNA and exhibit species- and cell type-specific features [6] , [7] , [8] . Chromatin architecture may have particular importance in neurons, because these long-living cells are permanently arrested in interphase and the structures formed during neuronal differentiation are probably irreversible [9] , [10] , [11] . During neuronal maturation, the nuclear architecture of neural precursors undergoes dramatic changes and passes from a small, heterochromatic nucleus with many small chromocenters to the large euchromatic nucleus with a few large chromocenters characteristic of mature neurons [12] . Although the functional consequences of these changes are obscure, the conserved pattern in terminally differentiated neurons suggests that they are physiologically relevant. For instance, studies in Purkinje neurons have revealed a precise assembly process in which specific chromosomes always cluster together and adjacent neurons have similar spatial distribution of centromeric and telomeric clusters [13] , [14] . Furthermore, recent studies have shown that gene mutations associated with intellectual disability in humans affect chromatin compactation and the number and size of chromocenters in cortical neurons [15] , [16] . The reported changes in the spatial distribution of satellite DNA and active loci in hippocampal neurons after seizures or experimentally induced long-term potentiation also support a role for higher-order chromatin structures in neuronal function [17] , [18] , [19] . Also consistent with this view, a recent study has revealed chromosomal conformation changes in the chromatin of the prefrontal cortex of schizophrenic patients that specifically affected the GAD1 locus [20] . Serendipitously, the generation of bitransgenic mice that express a histone H2B tagged with green fluorescent protein (H2BGFP) in an inducible manner in principal neurons of the forebrain provided us with an unexpected and valuable approach to examine the consequences of interfering with 3D chromatin organization in neuronal gene expression and physiology. We found that the accumulation of H2BGFP causes dramatic changes in the nuclear architecture of pyramidal neurons, including chromocenter declustering and loss of peripheral heterochromatin. These changes are accompanied by highly specific transcriptional defects and behavioural abnormalities, including alterations associated with serotonin (5-HT) dysfunction. Our results suggest a new role for perinuclear heterochromatin and chromocenter organization in the epigenetic regulation of neuronal gene expression that may have relevance in the aetiology of mental illness. Aberrant chromatin architecture in H2BGFP-expressing neurons To label the nucleus of principal neurons in the forebrain, we used the doxycycline (dox)-regulated system of double transgenics [21] to express a fusion protein between histone H2B and GFP ( Fig. 1a ). Double transgenics raised off dox expressed high levels of H2BGFP in principal neurons of the forebrain, particularly in the CA1 and DG subfields of the hippocampus, specific layers of the cortex and striatum ( Fig. 1b ). Reverse transcription–quantitative PCR (RT–qPCR) and western blot assays indicated that the chimeric histone is expressed at a comparable level to endogenous histone H2B and is functionally integrated into chromatin ( Fig. 1c–e ). Nissl staining and immunostaining for different neuronal proteins demonstrated that H2BGFP did not cause neuronal death nor gross alterations in brain anatomy ( Supplementary Fig. 1 ). 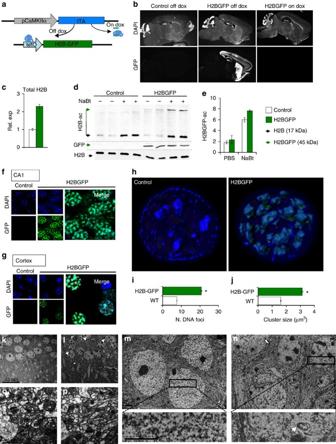Figure 1: Regulated expression of H2BGFP in the brain of transgenic mice is associated with aberrant DNA staining. (a) Bitransgenic approach used in this study. (b) GFP immunostaining of brain sagittal sections from H2BGFP mice, fed or not with dox, and a control littermate. DAPI was used for nuclear counterstaining. (c) qPCR assays using a primer pair that recognizes a highly conserved sequence present in both mouse and human H2B transcripts. (d) Western blot analyses using antibodies against H2Bac, GFP and H2B (top to bottom). H2BGFP was hyperacetylated similar to endogenous histone H2B after treatment with the inhibitor of histone deacetylases sodium butyrate (NaBt). (e) Relative intensity quantification of H2BGFP acetylation. (f,g) GFP and DAPI patterns in CA1 (f) and cortical (g) neurons of H2BGFP and control mice. (h) 3D reconstruction of confocal images illustrating both chromocenters declustering and the loss of peripheral heterochromatin in CA1 pyramidal neurons of H2BGFP mice. (i,j). Quantification of the number (i) and size (j) of DAPI-stained foci in H2BGFP and control littermates. (k–p) Electron micrographs of pyramidal neurons in the CA1 subfield of control (k) and H2BGFP mice (l). The higher magnification images of disorganized heterochromatin and insets illustrate the emptiness of nucleoplasm space and occasional presence of internal membranous structures in H2BGFP nuclei (n) compared with control littermates (m). In contrast, there is no apparent difference in the stratum radiatum of control (o) and H2BGFP mice (p). Figure 1: Regulated expression of H2BGFP in the brain of transgenic mice is associated with aberrant DNA staining. ( a ) Bitransgenic approach used in this study. ( b ) GFP immunostaining of brain sagittal sections from H2BGFP mice, fed or not with dox, and a control littermate. DAPI was used for nuclear counterstaining. ( c ) qPCR assays using a primer pair that recognizes a highly conserved sequence present in both mouse and human H2B transcripts. ( d ) Western blot analyses using antibodies against H2Bac, GFP and H2B (top to bottom). H2BGFP was hyperacetylated similar to endogenous histone H2B after treatment with the inhibitor of histone deacetylases sodium butyrate (NaBt). ( e ) Relative intensity quantification of H2BGFP acetylation. ( f , g ) GFP and DAPI patterns in CA1 ( f ) and cortical ( g ) neurons of H2BGFP and control mice. ( h ) 3D reconstruction of confocal images illustrating both chromocenters declustering and the loss of peripheral heterochromatin in CA1 pyramidal neurons of H2BGFP mice. ( i , j ). Quantification of the number ( i ) and size ( j ) of DAPI-stained foci in H2BGFP and control littermates. ( k – p ) Electron micrographs of pyramidal neurons in the CA1 subfield of control ( k ) and H2BGFP mice ( l ). The higher magnification images of disorganized heterochromatin and insets illustrate the emptiness of nucleoplasm space and occasional presence of internal membranous structures in H2BGFP nuclei ( n ) compared with control littermates ( m ). In contrast, there is no apparent difference in the stratum radiatum of control ( o ) and H2BGFP mice ( p ). Full size image In the course of these initial experiments, we observed that H2BGFP accumulated in discrete structures in the interior of the neuronal nucleus that were strongly labelled with the DNA stain 4',6-diamidino-2-phenylindole (DAPI). Although DAPI staining in the nucleus of CA1 neurons typically delineates the nuclear envelope and accumulates in a few large chromocenters, in bitransgenic animals DAPI fluorescence overlapped with GFP and provided a distinctive subnuclear pattern with numerous foci and without peripheral heterochromatin attached to the nuclear membrane ( Fig. 1f ). Similar but less pronounced differences were also observed in other neuronal types expressing H2BGFP, such as granular neurons in the dentate gyrus, and cortical and striatal neurons ( Fig. 1g ). Quantitative 3D analysis confirmed the increase in the number of intranuclear DAPI-stained foci in CA1 pyramidal neurons and revealed that these structures were larger and more irregular in bitransgenic than in control mice ( Fig. 1h–j and Supplementary Movies 1 and 2 ). To confirm these observations using a different approach that provides better spatial resolution, we used electron microscopy (EM). The comparison of EM images corresponding to the stratum pyramidale in the CA1 subfield revealed dramatic differences between H2BGFP and control littermates. In ultrathin sections, the nucleus of CA1 pyramidal neurons in control animals showed none or, at most, one to two heterochromatic regions ( Fig. 1k ), whereas bitransgenic mice exhibited multiple discrete heteropycnotic regions ( Fig. 1l ). Moreover, whereas the nuclei of control neurons show heterochromatin attached to the inner nuclear envelope, in H2BGFP mice this was detached (compare Fig. 1m,n ). In fact, some neurons in bitransgenic mice exhibited nuclear body-like circular membranous structures that may have originated from invaginations of the nuclear lamina during heterochromatin detachment. We also observed a reorganization of the interchromatin compartment, which appeared much emptier in H2BGFP mice than in control animals ( Fig. 1m,n , insets). These changes of nuclear ultrastructure did not alter the number or structure of synapses in the stratum radiatum ( Fig. 1o,p : Control=0.285 and H2BGFP=0.272 syn μm −2 ). To characterize the extent of the nuclear disorganization, we next conducted co-localization experiments with proteins or protein modifications that are known to be enriched in specific nuclear sub-structures. In agreement with EM images, the nucleolar proteins fibrillarin and nucleolin revealed that nucleoli were normal in H2BGFP-expressing neurons ( Fig. 2a ). The spliceosome protein Sam68 and the Cajal body protein coilin also revealed a normal staining pattern, indicating that these structures were preserved in bitransgenic mice ( Fig. 2b,c ). Lamina staining was also not affected, except for the occasional invaginations reported above ( Fig. 2d,e ). In contrast, fluorescence in situ hybridization (FISH) using a pancentromeric probe revealed striking differences between genotypes; in control nuclei the FISH signal overlapped with chromocenters, whereas in H2BGFP-expressing neurons the signal was scattered in the form of dots embedded within the aberrant DNA foci, in addition to some normal-looking chromocenters ( Fig. 2f ). H3K9me2/3 ( Fig. 2g ) and methyl-Cytosine (mCyt, Fig. 2h ), two modifications of the chromatin associated with a heterochromatic state, also exhibited an aberrant staining pattern that overlapped with GFP/DAPI foci. This redistribution was associated with a significant reduction of the signal for mCyt (Control=1.00±0.38, H2BGFP=0.7±0.03, P <0.0001). Interestingly, the expression of H2BGFP caused a shifting of the signal for the intercalating agent propidium iodide (PI) in flow cytometry experiments ( Fig. 2i ) that disappeared when the nuclei were pre-incubated with HCl to extract chromatin proteins and allow the full access of PI to DNA, which suggests that the accessibility to PI in a fraction of the chromatin is larger in H2BGFP-expressing neurons. Immunostaining for H3K27me3, a histone post-translational modification (PTM) that can be found in both active and inactive loci but not in silent chromatin, also revealed dramatic differences between genotypes. Whereas in control animals H3K27me3 showed a diffuse pattern that excluded the large chromocenters, in bitransgenics the signal partially overlapped with the aberrant DAPI foci ( Fig. 2j ). A similar but milder redistribution was also observed for the methyl CpG binding protein 2, a transcriptional repressor that binds methylated DNA sequences ( Fig. 2k ). Finally, the staining patterns for several protein modifications associated with euchromatin were also altered. Thus, whereas the staining for histone acetylations ( Fig. 2l ) and phospho-Pol II S5P ( Fig. 2j ) filled most of the nucleus in normal neurons, concentrating at brighter spots (possibly transcription factories), they accumulated around GFP/DAPI foci in bitransgenic mice. This accumulation was particularly pronounced in the case of H3K9ac that showed a striking ring-like pattern around the foci. Together, these results demonstrate that H2BGFP expression is associated with an abnormal interaction between heterochromatin and the nuclear lamina, the declustering of pericentromeric chromatin and the re-organization of transcriptionally active domains. 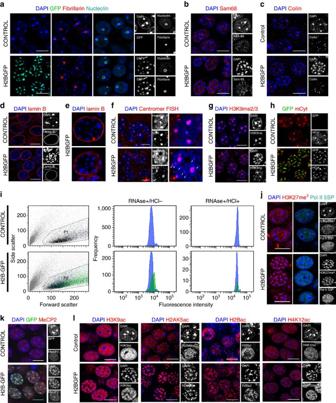Figure 2: H2BGFP expression alters heterochromatin and euchromatin organization in hippocampal CA1 neurons. (a) Quadruple fluorescent imaging of brain slices from control and H2BGFP mice detecting native GFP fluorescence, immunostaining for two nucleolar proteins (fibrilarin and nucleolin) and DNA counterstaining with DAPI. (b) Immunostaining against Sam68, a protein enriched at the splicesome, revealed no difference between control and H2BGFP mice. (c) Immunostaining against coilin, a protein located at Cajal bodies, revealed no difference. (d,e) Immunostaining with lamin B was normal in most cells (d), although a small percentage of H2BGFP-expressing neurons exhibited lamin B invaginations (e, arrows). (f) Pancentromeric probe FISH revealed the declustering of centromeres in H2BGFP mice. Note the association of centromere label with numerous DNA foci in bitransgenic mice (arrows). (g) Immunostaining of brain slices using antibodies against the heterochromatin-associated histone modification H3K9me2/3. (h) Double immunostaining using antibodies against GFP and mCyt. (i) Flow cytometry of H2BGFP nuclei from hippocampal cells. The difference in PI signal observed in GFP+cells disappeared on HCl treatment. (j) Double immunostaining using antibodies against H3K27me3 and phospho-pol II S5P. (k) Double immunostaining using antibodies against GFP and methyl CpG binding protein 2 (MeCP2). (l) Immunostaining against H3K9,14ac, H2AK5ac, pan-H2Bac and H4K12ac. Scale bars, 10 μm. Nuclei were counterstained with DAPI except when indicated otherwise. Figure 2: H2BGFP expression alters heterochromatin and euchromatin organization in hippocampal CA1 neurons. ( a ) Quadruple fluorescent imaging of brain slices from control and H2BGFP mice detecting native GFP fluorescence, immunostaining for two nucleolar proteins (fibrilarin and nucleolin) and DNA counterstaining with DAPI. ( b ) Immunostaining against Sam68, a protein enriched at the splicesome, revealed no difference between control and H2BGFP mice. ( c ) Immunostaining against coilin, a protein located at Cajal bodies, revealed no difference. ( d , e ) Immunostaining with lamin B was normal in most cells ( d ), although a small percentage of H2BGFP-expressing neurons exhibited lamin B invaginations ( e , arrows). ( f ) Pancentromeric probe FISH revealed the declustering of centromeres in H2BGFP mice. Note the association of centromere label with numerous DNA foci in bitransgenic mice (arrows). ( g ) Immunostaining of brain slices using antibodies against the heterochromatin-associated histone modification H3K9me2/3. ( h ) Double immunostaining using antibodies against GFP and mCyt. ( i ) Flow cytometry of H2BGFP nuclei from hippocampal cells. The difference in PI signal observed in GFP + cells disappeared on HCl treatment. ( j ) Double immunostaining using antibodies against H3K27me3 and phospho-pol II S5P. ( k ) Double immunostaining using antibodies against GFP and methyl CpG binding protein 2 (MeCP2). ( l ) Immunostaining against H3K9,14ac, H2AK5ac, pan-H2Bac and H4K12ac. Scale bars, 10 μm. Nuclei were counterstained with DAPI except when indicated otherwise. Full size image Interference with heterochromatin structures Previous studies indicate that H2BGFP does not interfere with most chromatin functions in dividing cells, including transcription and mitosis [22] . Our results, however, show that the continuous and robust expression of this chimeric histone can destabilize heterochromatin structures in the quiescent nuclei of forebrain neurons. The modelling of nucleosomes bearing H2BGFP instead of H2B indicates that the bulky GFP tag (a barrel with radius and height of ~30 Å) will prominently protrude from the chromatin fibre and may interfere with the folding of the chromatin fibre in highly compacted tertiary structures ( Fig. 3a ), such as the dense interdigitation of nucleosomal arrays that has been postulated as a possible arrangement for heterochromatin in vivo [23] . 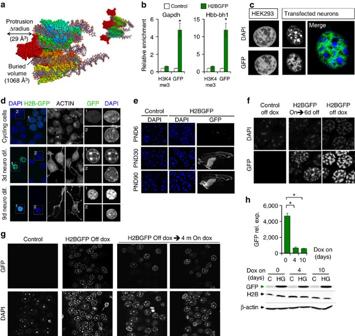Figure 3: H2BGFP accumulation destabilizes highly compacted chromatin structures. (a) Model of nucleosome sandwich incorporating a single H2BGFP molecule (in red). The steric difficulty to accommodate the GFP tag increases if we consider that each nucleosome may contain up to two molecules of GFP (upper right inset). (b) ChIP assays using anti-GFP antibody indicate that H2BGFP is incorporated into chromatin and enriched in silent genes. Data are represented as mean±s.e.m.;n=9 for both genotypes in H3K4me3 analysis;n=4 (control) and 5 (H2BGFP) in GFP analysis; *P<0.05. (c) HEK293 cells and primary hippocampal neurons (10 DIV) 24 h after transfection with a H2BGFP-expressing construct show normal DNA staining. (d) Neuro-2a cells were transfected with an H2BGFP-expressing construct and then treated with dbcAMP to stop proliferation and promote neuronal differentiation. H2BGFP expression was associated with progressive loss of chromatin architecture in differentiating cells (pictures correspond to 3 and 9 days after adding dbcAMP to the medium). (e) At postnatal day 6 (PND6), CA1 neurons of bitransgenic mice express very low or no GFP and exhibit a normal intranuclear organization. At PND30, CA1 neurons of bitransgenic mice express strong GFP fluorescence and show the same aberrant pattern described for adult mice (PND90). (f) Induction of transgene expression in adult mice triggers a progressive disruption of chromocenter organization. (g) GFP expression is still detected in the nucleus of CA1 neurons in H2BGFP mice 4 months after dox addition to the mouse diet. Note that the neurons that do not express GFP fluorescence have recovered a normal DNA staining pattern with few large chromocenters and peripheral heterochromatin. Images correspond to 9-month-old mice that were either kept out of dox (Control and H2BGFP Off dox images) or in which dox was added to the diet when the animals were 5 months old. The two sets of images under the ‘H2BGFP Off dox * 4 m On dox’ label correspond to two independent animals. (h). RT–qPCR (up) and western blot (down) assays indicates that although RNA levels were severely reduced in mice fed with dox for 4 or 10 days, protein levels were not reduced. Data are represented as mean±s.e.m.;n=2 per group; *P<0.05. Figure 3: H2BGFP accumulation destabilizes highly compacted chromatin structures. ( a ) Model of nucleosome sandwich incorporating a single H2BGFP molecule (in red). The steric difficulty to accommodate the GFP tag increases if we consider that each nucleosome may contain up to two molecules of GFP (upper right inset). ( b ) ChIP assays using anti-GFP antibody indicate that H2BGFP is incorporated into chromatin and enriched in silent genes. Data are represented as mean±s.e.m. ; n =9 for both genotypes in H3K4me3 analysis; n =4 (control) and 5 (H2BGFP) in GFP analysis; * P <0.05. ( c ) HEK293 cells and primary hippocampal neurons (10 DIV) 24 h after transfection with a H2BGFP-expressing construct show normal DNA staining. ( d ) Neuro-2a cells were transfected with an H2BGFP-expressing construct and then treated with dbcAMP to stop proliferation and promote neuronal differentiation. H2BGFP expression was associated with progressive loss of chromatin architecture in differentiating cells (pictures correspond to 3 and 9 days after adding dbcAMP to the medium). ( e ) At postnatal day 6 (PND6), CA1 neurons of bitransgenic mice express very low or no GFP and exhibit a normal intranuclear organization. At PND30, CA1 neurons of bitransgenic mice express strong GFP fluorescence and show the same aberrant pattern described for adult mice (PND90). ( f ) Induction of transgene expression in adult mice triggers a progressive disruption of chromocenter organization. ( g ) GFP expression is still detected in the nucleus of CA1 neurons in H2BGFP mice 4 months after dox addition to the mouse diet. Note that the neurons that do not express GFP fluorescence have recovered a normal DNA staining pattern with few large chromocenters and peripheral heterochromatin. Images correspond to 9-month-old mice that were either kept out of dox (Control and H2BGFP Off dox images) or in which dox was added to the diet when the animals were 5 months old. The two sets of images under the ‘H2BGFP Off dox * 4 m On dox’ label correspond to two independent animals. ( h ). RT–qPCR (up) and western blot (down) assays indicates that although RNA levels were severely reduced in mice fed with dox for 4 or 10 days, protein levels were not reduced. Data are represented as mean±s.e.m. ; n =2 per group; * P <0.05. Full size image Based on this observation and the previous evidence indicating that H2BGFP molecules are rapidly exchanged in active nucleosomes during transcription but retained in non-active chromatin domains [24] , we speculate that this chimeric histone would progressively accumulate into heterochromatin, sterically destabilizing the highly compacted tertiary chromatin structures characteristic of fully differentiated neurons. Consistent with this view, the relative enrichment for H2BGFP in hippocampal chromatin at steady state was larger in silent genes, such as Hbb-bh1 , than in highly expressed genes, such as Gapdh ( Fig. 3b ). In addition, supporting the specificity of the effect of chronic H2BGFP expression in neuronal nuclear architecture, we found that H2BGFP did not alter DAPI staining in HEK293 cells or transiently transfected cultured hippocampal neurons ( Fig. 3c ). Most glial cells in bitransgenic mice generated by crossing tetO-H2BGFP mice with pGFAP-tTA also showed a normal DNA distribution ( Supplementary Fig. 2 ). In contrast, neural crest-derived Neuro-2a cells transfected with H2BGFP appeared initially normal but exhibited an aberrant chromatin distribution after dibutyryl-cAMP-induced differentiation to a neuronal phenotype ( Fig. 3d ). The latter experiment also revealed a good correlation between the level of H2BGFP expression and the strength of the chromatin phenotype. Additional experiments in transgenic mice demonstrated that chromocenter declustering closely correlated with transgene expression. Thus, the neurons of 6-day-old bitransgenic mice, in which transgene expression was nearly undetectable, exhibited a normal nuclear pattern with few large chromocenters, whereas 3 weeks later young bitransgenic animals already presented the aberrant staining described for adult mice ( Fig. 3e ). On the other hand, bitransgenic mice raised on a dox-supplemented diet did not express the transgene and exhibited normal DAPI staining ( Fig. 1b , right panels), but incipient chromocenter disorganization became evident 1 week after transgene induction and was completed 2 weeks later ( Fig. 3f ). Consistently, transgene repression by continuous treatment with dox for several months led to the appearance of scattered neurons that showed the loss of both GFP fluorescence and the aberrant DAPI staining phenotype ( Fig. 3g ). Note that the very long half-life of this protein [25] caused that the rapid decrease of H2BGFP transcripts by dox was not followed by a similar reduction at the protein level ( Fig. 3h ). Loss of chromatin architecture and transcription We next investigated the consequences of aberrant chromatin organization in global gene expression using microarrays. This analysis revealed that the dramatic structural changes had a surprisingly modest impact on hippocampal gene expression ( Fig. 4a ). Heterochromatin disorganization did not cause the de-repression of non-neuronal genes or transcriptionally repressed repetitive elements. In fact, most of the detected changes corresponded to genes downregulated in H2BGFP mice ( Fig. 4b and Supplementary Table 1 ). The differential profiling retrieved transcript cluster IDs of particular relevance for neuronal function and behaviour, such as Drd5 , Npy2r , Htr1a , Htr1b and Htr2a that encode for a dopamine, a neuropeptide and three serotonin receptors, respectively. Indeed, negative regulation of glutamatergic synaptic transmission (adj. P =7 × 10 −5 ), serotonin receptor signalling (adj. P =1 × 10 −4 ) and dopamine secretion (adj. P =2 × 10 −4 ) were the most affected biological processes in the H2BGFP profile according to Gene Ontology analysis ( Supplementary Table 2 ). The functional analysis also revealed a significant association with abnormal anxiety-related response (adj. P =3 × 10 −4 ), abnormal spatial learning (adj. P =6 × 10 −4 ), abnormal locomotor activation (adj. P =5 × 10 −3 ) phenotypes and a number of disturbances of the conduct in humans that included attention deficit disorder with hyperactivity (adj. P =2 × 10 −7 ) and other behavioural disorders (adj. P <1 × 10 −6 ). 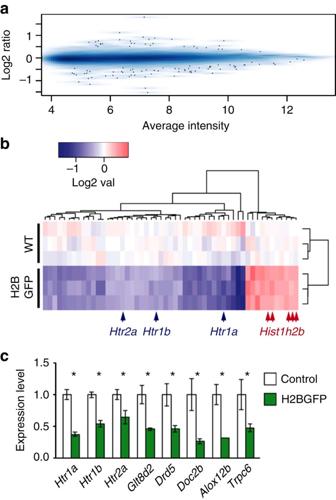Figure 4: Transcriptional dysregulation in H2BGFP mice. (a) MA plot summarizing differential expression in H2BGFP mice. (b) Heatmap showing the top 50 TCIDs differentially expressed in H2BGFP mice. Gene downregulations (blue) were much more abundant than upregulations (red); several upregulated TCIDs recognizes histone H2B transcripts and probably report transgene expression. (c) Biological validation of candidate genes by RT–qPCR analysis. *P<0.05 (Student’st-test),n=5 per group. Figure 4: Transcriptional dysregulation in H2BGFP mice. ( a ) MA plot summarizing differential expression in H2BGFP mice. ( b ) Heatmap showing the top 50 TCIDs differentially expressed in H2BGFP mice. Gene downregulations (blue) were much more abundant than upregulations (red); several upregulated TCIDs recognizes histone H2B transcripts and probably report transgene expression. ( c ) Biological validation of candidate genes by RT–qPCR analysis. * P <0.05 (Student’s t -test), n =5 per group. Full size image RT–qPCR assays using independent samples confirmed the most relevant transcriptional changes, including the downregulation of 5-HT receptors ( Fig. 4c ), and the absence of significant changes in repetitive elements ( Supplementary Fig. 3a ). Behavioural abnormalities in H2BGFP mice We next examined whether animal’s behaviour was affected as predicted by our functional analysis of differential expression. No differences were observed between bitransgenic mice and control siblings in a battery of neurological tests assessing basic reflexes, strength and other parameters ( Supplementary Table 3 ). Motor performance in an accelerated Rotarod task was also not affected ( Supplementary Fig. 4a : F (1, 16) genotype =0.10, P =0.75). However, bitransgenic mice showed locomotor hyperactivity in an open arena measured as ambulatory distance ( Fig. 5a : F (1, 16) genotype =24.92, P =0.0001; see also Supplementary Fig. 4b ), reduced resting time ( Fig. 5b : F (1, 16) genotype =24.46, P =0.0001) and faster speed ( Fig. 5c : F (1, 16) genotype =23.46, P =0.0002). Bitransgenic mice also presented deficits in tasks evaluating their responsiveness to different sort of external stimuli, including reduced marble burying behaviour ( Fig. 5d : F (1, 16) genotype =10.67, P =0.005), larger latencies for exploring novel objects ( Fig. 5e : F (1, 16) genotype =7.87, P =0.01), impaired social interaction ( Fig. 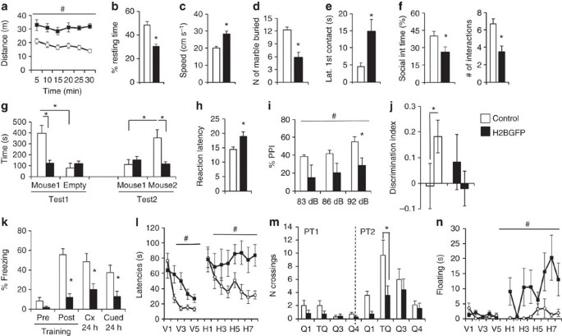Figure 5: Behavioural consequences of the loss of chromatin architecture. (a–c) Total travelled distance (a), resting time (b) and speed (c) in an open arena. (d) Performance in the marble burring task. (e) Time taken to first approach a novel object in a familiar arena. (f) Performance in social interaction task. (g) Performance in the three-chambered social approach task (Test1), and social novelty preference task (Test2). (h) Latency for first reaction in the hot plate test. (i) Performance in the Prepulse inhibition (PPI) test. (j) Performance in the NOR task. (k) Performance in the fear-conditioning task. (l–n) Visible and hidden platform watermaze tasks: latency to find the platform (l); number of crossing in the two probe trials (PT1 and PT2) (m); and time floating (n). TQ, target quadrant;#genotype effect<0.05 (repeated-measure analysis of variance); *P<0.05. (a–h):n=9, both groups; (i): 8 control and 7 H2BGFP; (j,k): 9 control and 7 H2BGFP; (l–n):n=7, both groups. H2BGFP: dark squares; control: open circles. SeeSupplementary Fig. 4for additional details. 5f : F (1, 16) genotype =5.42, P =0.03; Figure 5g : F (1, 16) genotype =0.44, P =0.02), larger latencies in the hot plate task ( Fig. 5h : F (1, 16) genotype =6.64, P =0.02) and deficits in sensorimotor gating ( Fig. 5i : F (1, 13) genotype =6.06, P =0.03), but normal startle response ( Supplementary Fig. 4c : F (1, 13) genotype =0.12, P =0.73). Figure 5: Behavioural consequences of the loss of chromatin architecture. ( a – c ) Total travelled distance ( a ), resting time ( b ) and speed ( c ) in an open arena. ( d ) Performance in the marble burring task. ( e ) Time taken to first approach a novel object in a familiar arena. ( f ) Performance in social interaction task. ( g ) Performance in the three-chambered social approach task (Test1), and social novelty preference task (Test2). ( h ) Latency for first reaction in the hot plate test. ( i ) Performance in the Prepulse inhibition (PPI) test. ( j ) Performance in the NOR task. ( k ) Performance in the fear-conditioning task. ( l – n ) Visible and hidden platform watermaze tasks: latency to find the platform ( l ); number of crossing in the two probe trials (PT1 and PT2) ( m ); and time floating ( n ). TQ, target quadrant; # genotype effect<0.05 (repeated-measure analysis of variance); * P <0.05. ( a – h ): n =9, both groups; ( i ): 8 control and 7 H2BGFP; ( j , k ): 9 control and 7 H2BGFP; ( l – n ): n =7, both groups. H2BGFP: dark squares; control: open circles. See Supplementary Fig. 4 for additional details. Full size image H2BGFP mice were also impaired in several cognitive tasks. We should, however, note that the existence of underlying basic behavioural alterations, such as hyperlocomotion in the open field and reduced nociception, prevents a precise evaluation of cognitive capabilities. In the novel object recognition (NOR) task, control mice spent more time exploring a novel than a familiar object ( Fig. 5j : F (1, 8) =1.93, P =0.05), whereas H2BGFP mice spent similar time in exploring both objects, showing no memory for previously explored objects ( F (1, 6) =0.93, P =0.37). Similarly, bitransgenic mice did not express a preference for interacting with a novel versus a previously encountered mouse in the three-chambered social novelty task ( Fig. 5g : F (1, 16) genotype =0.47, P =0.02). H2BGFP mice also exhibited significant deficits in contextual ( Fig. 5k : F (1, 14) genotype =7.31, P =0.02) and cued ( F (1, 14) genotype =6.16, P =0.03) fear conditioning, and a reduced immediate response to the shock ( F (1, 14) genotype =33.0, P <0.001). Furthermore, in the hidden platform water maze task, H2BGFP mice showed severe deficits in spatial learning manifested in the latency ( Fig. 5l : F (7, 84) time × genotype =1.89, P =0.04) and path length ( Supplementary Fig. 4d : F (7, 84) time × genotype =2.95, P =0.008) curves that led to very poor performance in the probe trials assessing spatial memory ( Fig. 5m : PT1 TQ F (1, 12) =1.96, P =0.19; PT2 TQ F (1, 12) =5.13, P =0.04; see also Supplementary Fig. 4e ). Importantly, these mice also swam slower ( Supplementary Fig. 4f : F (1, 12) genotype =5.44, P =0.04) and, starting after the visible platform task, were more prone to floating ( Fig. 5n : F (7, 84) time × genotype =2.39, P =0.03), which is consistent with the reduced responsiveness observed in other tasks. These behavioural deficits are probably not caused by a failure in activity-driven transcription because the well-characterized and transient induction of immediate early genes on novelty exposure, which includes genes involved in neuronal plasticity and memory consolidation such as Fos , Arc and Npas4 (ref. 26 ), was preserved in the hippocampus of H2BGFP mice despite of the severe chromatin disorganization ( Supplementary Fig. 3b ). Epigenetic dysregulation of serotonin receptor genes Prompted by our functional analysis of differential gene expression, we examined in detail the genomic features of behaviourally relevant loci whose expression was altered in H2BGFP mice. We observed that the three 5-HT receptor genes downregulated in bitransgenic mice ( Htr1a , Htr1b and Htr2a ) had, in common, their location adjacent to desert islands ( Fig. 6a,b ). The examination of the hippocampal profiles for H3K4me3 and H3K9,14ac recently generated by our group [27] confirmed the large distance between these loci and the nearest active gene in hippocampal tissue ( Fig. 6c ). Consistently, the exploration of the profiles recently generated by Ren’s lab in their screen for cis -regulatory sequences in the mouse cerebral cortex [28] did not identify any prominent putative regulatory element in these genomic regions ( Supplementary Fig. 5a ). The comparison with the same region in the human genome reveals high synteny and conserved spacing between the two species. Other genes at the edge of gene desert, such as Fat4 , Gpr101 and Ptpru , were also downregulated in H2BGFP mice. Overall, 13% of the genes in which the distance to one of its two neighbours is >0.5 Mbp (660 genes, 59% of them showing an expression in hippocampal tissue higher than the median) where altered in H2BGFP mice (Fisher’s exact test P -value=0.01). The significance of this enrichment is even larger if we consider a neighbour distance >250 Kb ( P -value=1.8 × 10 −5 ). The position of these genes in the interphase between euchromatin and heterochromatin might contribute to explain their larger susceptibility to changes in chromatin architecture, although additional gene features should lend specificity to this sensitivity, because not all the genes located in the proximity of gene-free regions were affected by H2BGFP expression. 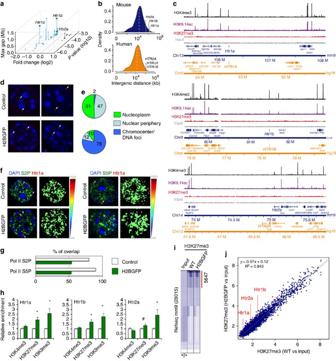Figure 6: Epigenetic dysregulation of serotonin receptor genes. (a) Plot presenting the fold change,P-value and distance to farthest neighbour of genes inFig. 4b. (b) The distance betweenHtr1a,Htr1bandHtr2a, and, at least, one of the two adjacent genes is far above the median, both in mice (blue) and humans (orange). (c) Genomic view of theHtr1a,Htr1bandHtr2aloci in the mouse (blue) and human (orange) genome, and the profiles in hippocampal chromatin for H3K4me3 and H3K9,14ac and H3K27me3 histone marks. (d) FISH forHtr1a(red, arrow heads) with Hoechst counterstaining. The sector graphs show the percentage ofHtr1aalleles located at the nuclear periphery, associated with chromocenter/internal DNA foci or the nucleoplasm. (e,f) Association ofHtr1aalleles (red, arrow heads) with the activated forms of Pol II S2P (e) and S5P (f), both labelled in green. Colour maps represent the correlation coefficient between intensities of Pol II signal and hybridization signal. (g) Quantification of the experiments ineandf. (h) ChIP assays at theHtr1a,Htr1bandHtr2apromoters. Data are represented as mean±s.e.m.;n=3 per group; *P<0.05;#P=0.07. (i) Heatmap of read densities across Refseq TSSs (10 kb window around TSS) in input and H3K27me3 data sets. Red bar: 5,647 genes. (j) Scatter plot of H3K27me3 enrichment in the hippocampus of H2BGFP and control mice. The regression line (green dotted line) and coefficient of determination are shown. Figure 6: Epigenetic dysregulation of serotonin receptor genes. ( a ) Plot presenting the fold change, P -value and distance to farthest neighbour of genes in Fig. 4b . ( b ) The distance between Htr1a , Htr1b and Htr2a , and, at least, one of the two adjacent genes is far above the median, both in mice (blue) and humans (orange). ( c ) Genomic view of the Htr1a , Htr1b and Htr2a loci in the mouse (blue) and human (orange) genome, and the profiles in hippocampal chromatin for H3K4me3 and H3K9,14ac and H3K27me3 histone marks. ( d ) FISH for Htr1a (red, arrow heads) with Hoechst counterstaining. The sector graphs show the percentage of Htr1a alleles located at the nuclear periphery, associated with chromocenter/internal DNA foci or the nucleoplasm. ( e , f ) Association of Htr1a alleles (red, arrow heads) with the activated forms of Pol II S2P ( e ) and S5P ( f ), both labelled in green. Colour maps represent the correlation coefficient between intensities of Pol II signal and hybridization signal. ( g ) Quantification of the experiments in e and f . ( h ) ChIP assays at the Htr1a , Htr1b and Htr2a promoters. Data are represented as mean±s.e.m. ; n =3 per group; * P <0.05; # P =0.07. ( i ) Heatmap of read densities across Refseq TSSs (10 kb window around TSS) in input and H3K27me3 data sets. Red bar: 5,647 genes. ( j ) Scatter plot of H3K27me3 enrichment in the hippocampus of H2BGFP and control mice. The regression line (green dotted line) and coefficient of determination are shown. Full size image We next investigated the association of the most affected and clinically relevant of these loci, Htr1a , with peripheral heterochromatin and chromocenters through FISH. Consistently with a recent screen for lamina-associated domains ( Supplementary Fig. 5b ), quantitative FISH analysis of Htr1a in control animals revealed a non-random spatial distribution in the nucleus of CA1 neurons, in which one of the two Htr1a alleles was frequently positioned at the nuclear margin, whereas the other was at the nucleus interior ( Fig. 6d and Supplementary Fig. 6 ). This configuration was altered in neurons from H2BGFP mice, in which in the absence of perinuclear heterochromatin, the two Htr1a alleles were positioned in the proximity of, or even within, the aberrant DNA-foci ( Fig. 6d and Supplementary Fig. 6 , note that Htr1a signal is consistently associated with the less bright foci originated after chromocenter declustering.). To assess the functional status of the locus, we performed immuno-FISH assays to simultaneously detect the Htr1a alleles and activated RNA polymerase II phospho-epitopes p-Ser2 or p-Ser5 ( Fig. 6e,f ). In agreement with our gene expression data, the quantitative analysis revealed that the association of Htr1a with these two phosho-proteins was larger in control than in H2BGFP mice ( Fig. 6g : Control S2P=89±1.0%, H2BGFP S2P=53±0.9%; Control S5P=79±1.0%, H2BGFP S5P=53±0.8%). Moreover, the reduced expression and intranuclear relocation was associated with the spreading of heterochromatin PTMs into this locus ( Fig. 6h ). Also consistently with gene expression data, similar results were obtained at the promoters of Htr1b and Htr2a ( Fig. 6h ). In our effort to investigate the relationship between the global changes in chromatin architecture and the, in contrast, highly specific transcriptional changes, we determined the genomic profile of H3K27me3 in the chromatin of H2BGFP mice and control littermates. This histone PTM is found at the boundaries of lamin-bound domains and has been traditionally considered a repressive chromatin mark, although is mutually exclusive with H3K9 methylation. Although the intranuclear (3D) distribution of H3K27me3 is severely disrupted by H2BGFP expression ( Fig. 2j ), chromatin immunoprecipitation sequencing (ChIP-seq) analysis did not reveal dramatic alterations of its (two-dimensional) genomic profile ( Fig. 6i and Supplementary Fig. 7a ). Notably, the genomic screen confirmed the increase of H3K27me3 presence in Htr loci detected in locus-specific assays ( Fig. 6j ) but did no reveal any major change in the topography of this mark neither in the loci nor in the adjacent gene desert regions ( Fig. 6c and Supplementary Fig. 7b ). As expected from studies outside the brain, the larger enrichment for H3K27me3 was found in developmental homeobox genes silenced in adult tissue ( Supplementary Fig. 7c ). To determine whether serotonin signalling was effectively reduced in H2BGFP-expressing CA1 pyramidal neurons, we performed electrophysiological recordings in CA1 pyramidal neurons of bitransgenic and control littermates. Serotonin binding to 5-HT 1A subtype receptors (encoded by Htr1a ) in the membrane of CA1 neurons activates G protein-coupled inwardly rectifying K + channels causing cell hyperpolarization and the reduction of membrane resistance [29] , [30] . Both parameters were significantly reduced in the neurons of bitransgenic animals after serotonin application ( Fig. 7a,b ). Moreover, the administration of the partial agonist of 5-HT 1A receptors buspirone, which modulates locomotor activity in the open field ( Fig. 7c : F (1, 30) drug treatment =10.31, P =0.003), restored the mobility of bitransgenic mice to control levels and increased the percentage of time that the mice spent interacting with a stranger mouse and the duration of social contacts in the social interaction task ( Fig. 7d,e ). These results indicate that some of the behavioural alterations revealed in our comprehensive screen are related to serotonergic dysfunction. 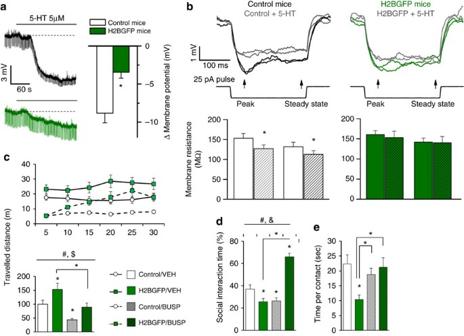Figure 7: Serotonin signalling is impaired in H2BGFP mice. (a) Effect of the application of 5 μM 5-HT on the resting membrane potential of CA1 pyramidal neurons from a control (black trace) or a H2BGFP (green trace) mouse. Dashed lines indicate the resting membrane potential (Control=−64.4±1.4 mV,n=10; H2BGFP=−63.8±1.4 mV,n=7;P=0.77). The bar graph shows the average hyperpolarization caused by 5-HT (*P=0.005,n=10 control, 7 H2BGFP). (b) Representative responses to 25 pA hyperpolarizing current pulses. Bar graphs show the average values of membrane input resistance in control (n=10,p(peak)=0.002,p(steady state)=0.007) and H2BGFP neurons (n=7, nonsignificant) treated (hatched bars) or not (open bars) with in 5-HT, at the peak of the hyperpolarizing response and at the end of the pulse (arrows). (c) Locomotor activity in an open arena (8 mice per group;#genotype effect<0.05;$drug effect<0.05). (d,e) Interaction time (e) and duration of social contacts (d) in a social interaction task (n=12 for vehicle (VEH),n=13 for buspirone (BUSP) groups;#genotype effect<0.05;$drug effect;&drug × genotype interaction<0.05); *P<0.05, Studentt-test comparison with control group at least that indicated otherwise. Figure 7: Serotonin signalling is impaired in H2BGFP mice. ( a ) Effect of the application of 5 μM 5-HT on the resting membrane potential of CA1 pyramidal neurons from a control (black trace) or a H2BGFP (green trace) mouse. Dashed lines indicate the resting membrane potential (Control=−64.4±1.4 mV, n =10; H2BGFP=−63.8±1.4 mV, n =7; P =0.77). The bar graph shows the average hyperpolarization caused by 5-HT (* P =0.005, n =10 control, 7 H2BGFP). ( b ) Representative responses to 25 pA hyperpolarizing current pulses. Bar graphs show the average values of membrane input resistance in control ( n =10, p (peak) =0.002, p (steady state) =0.007) and H2BGFP neurons ( n =7, nonsignificant) treated (hatched bars) or not (open bars) with in 5-HT, at the peak of the hyperpolarizing response and at the end of the pulse (arrows). ( c ) Locomotor activity in an open arena (8 mice per group; # genotype effect<0.05; $ drug effect<0.05). ( d , e ) Interaction time ( e ) and duration of social contacts ( d ) in a social interaction task ( n =12 for vehicle (VEH), n =13 for buspirone (BUSP) groups; # genotype effect<0.05; $ drug effect; & drug × genotype interaction<0.05); * P <0.05, Student t -test comparison with control group at least that indicated otherwise. Full size image We demonstrate here that the robust expression of histone H2B tagged with enhanced GFP in mature neurons causes a dramatic reorganization of chromatin that affected the association of heterochromatin with the nuclear lamina, the higher-order organization of pericentromeric heterochromatin in large chromocenters that is characteristic of mature cortical and hippocampal pyramidal neurons, and the subnuclear distribution of protein PTMs associated with active transcription. Although GFP-tagged histones are a common tool in cellular and developmental biology studies, our experiments indicate that caution is needed while using this tool in studies of the adult brain. Two unique features of our study led to this finding. First, most previous studies with GFP-tagged histone H2B have been performed after transient expression and/or in dividing cell, whereas we investigated the quiescent postmitotic nuclei of mature pyramidal neurons at the steady state. Second, the aberrant DAPI pattern was first noted in mouse CA1 hippocampal neurons, which have a particularly prominent and characteristic chromocenter organization. In differentiated cells, chromatin is spatially segregated in different types [5] . Chromocenters and peripheral heterochromatin represent the highest level of chromatin compactation and are labelled with epigenetic modifications associated with silent DNA (for example, mCyt and H3K9me2/3), whereas transcriptionally active domains are located in the nucleoplasm and enriched in histone modifications associated with an open chromatin conformation, such as the acetylation of histone tails and H3K4me3. This spatial configuration is profoundly disturbed by H2BGFP, possibly as a result of its shuttling in active chromatin and retention in non-active domains where it sterically interferes with highly compacted heterochromatin conformations. These changes also affected less compacted forms of chromatin and, as a result, the characteristic dispersed pattern of H3K27me3 in interphase nuclei was replaced in bitransgenic mice by a patched pattern that overlapped with GFP/DAPI foci (although in the absence of apparent changes in its genomic distribution), whereas histone PTMs associated with active transcription clustered in the surface of these structures. Notably, other subnuclear structures, such as the nucleolus or the Cajal bodies, were not affected by these changes of nuclear architecture. Taken together, our results indicate that the loss of one heterochromatin compartment has a broad impact on chromatin compartmentalization and highlight the fine interplay between histone PTMs that regulate the transition between different chromatin configurations [31] . The dramatic changes in chromatin architecture had a surprisingly subtle impact in gene expression. This observation indicates that either H2BGFP causes some specific transcriptional alterations that mediate the changes in chromatin distribution or, more probably, H2BGFP induces an aberrant chromatin conformation that leads to the transcriptional deregulation of specific loci. Given that none of the genes affected in H2BGFP mice is known to play a major role in chromatin organization, whereas H2BGFP is an integrant component of the chromatin in these neurons that has the potential to severely disrupt its packaging, we favour the second hypothesis. Intriguingly, the short list of genes affected by H2BGFP expression was enriched in genes that are adjacent to gene-free genomic regions. The large chromocenters in fully differentiated pyramidal neurons might represent the ultimate storage solution for DNA that will no longer be replicated nor transcribed. Our results suggest that the functional state of this inert DNA did not change as a result of chromocenter destabilization, but its decompaction and the concurrent relocation of active domains in the surface of the DNA foci observed in our co-staining experiments ( Fig. 2 ) may be responsible for the reduction in the transcription of active genes that are located in its immediate proximity. However, additional gene features should lend specificity to this epigenetic inactivation because not all the genes located in the proximity of gene-free regions were affected by H2BGFP expression. Future genome-wide chromosome conformational capture experiments might clarify this issue and relate specific changes in gene clustering to the transcriptional deficits reported here. Our study complements recent research demonstrating that intellectual disability disorders in humans are frequently associated with mutations in genes encoding chromatin regulators [32] and recent studies linking high-order chromatin organization and brain disease [19] , [20] , contributing to a better understanding of the still obscure role of chromatin architecture in brain function and gene expression. It allows to discern for the first time between processes that depend, or not depend, on such organization. Thus, our results indicate that 3D chromatin organization is not essential for neuronal viability or to maintain neuronal identity, but also show that its loss triggers physiological and behavioural deficits that are reminiscent of endophenotypes found in important behavioural disorders in humans. Furthermore, our experiments identified specific misregulated genes probably involved in these behavioural alterations. In particular, the changes in 5-HT1A receptor expression are considered an important determinant of predisposition to mental illness [33] and, although the mechanisms underlying the variable expression of this locus between individuals remain unclear, transcriptional dysregulation has been suggested as a probable candidate [34] . 5-HT2A and 5-HT1B receptors are also of great relevance for behavioural disorders [35] , [36] . These three 5-HT receptors are particularly abundant in corticolimbic regions targeted for H2BGFP expression in bitransgenic animals. Intriguingly, additional loci associated with mental illness, such as DRD5 and TDO2 , are also affected in H2BGFP mice. Both Drd5 (encoding for a dopamine receptor) and Tdo2 (encoding for the rate-limiting enzyme in the synthesis of serotonin tryptophan 2,3-dioxygenase) play a role in serotonin signalling and have been related to attention deficit-hyperactivity disorder and autism spectrum disorder [37] , [38] , [39] , [40] . The case of Rett syndrome (RS) is particularly interesting because (i) this congenital disorder associated with intellectual disability and autism has been recently related to impaired heterochromatin clustering [15] and chromocenter alterations during neuronal maturation [16] ; (ii) RS is caused by mutations in the gene encoding methyl CpG binding protein 2, one of the proteins showing abnormal distribution in H2BGFP-expressing neurons; (iii) the dysfunction of monoaminergic systems is known to be an important component of RS neuropathology [41] and 5-HT1A agonists, such as the one used in our study, prolong the life of mouse model of the disease [42] and are useful in the treatment of respiratory dysfunction in RS patients [43] ; and (iv) recent transcriptomics analyses show that Htr1a and Htr2a are downregulated in the hippocampus of mouse models of RS [44] . The transcriptional and behavioural deficits in H2BGFP mice also relate to negative symptoms in schizophrenia, such as prepulse inhibition and cognitive impairments, and reduce motivational drive. In fact, it has been proposed that alterations in serotonergic activity could be responsible for the dysregulation of dopaminergic function observed in schizophrenia, and some of the receptors downregulated in H2BGFP mice are found to be decreased in the prefrontal cortex of schizophrenia subjects as well [45] . We should, however, note that other relevant aspects of behaviour related to serotonin dysfunction, such as despair ( Supplementary Fig. 4g–h ) and anxiety ( Supplementary Fig. 4i–k ), were not altered in H2BGFP mice. The distinct actions of auto- and heteroreceptors [46] , and differential impact of impaired 5-HT signalling in immature and mature mood-related circuitry [47] , [48] together with the spatial and temporal pattern of transgenic expression, which restricts H2BGFP to areas of high heteroreceptor expression and late developmental stages, may explain the selective impact. Although it is unlikely that the disorganization of higher-order chromatin structure is a widespread feature of neuropsychiatric disorders, the overlap between the transcriptional deficits found in H2BGFP mice and some gene associations in neuropsychiatric disorders is striking. Our syntheny analysis revealed that the genes encoding the serotonin receptors affected in H2BGFP mice are also located in the proximity of gene deserts in humans. It is, therefore, attractive to speculate that this topographic feature may underlie a larger susceptibility of the loci to epigenetic regulation in response to experience and environmental changes. Animals and treatments pCaMKII-tTA/line B [21] and tetO-HIST1H2BJ/GFP [25] mice were crossed to produce CaMKII-tTA/tetO-H2BGFP bitransgenic mice that are referred to as ‘H2BGFP mice’ in the text. Both parental strains are available at Jackson Laboratories (stock number 7004 and 5104, respectively) and are maintained on a C57BL/6J genetic background (the second one after backcrossing to this background). H2BGFP mice were usually raised without dox and transgene repression was achieved by dox administration (40 mg kg −1 of food) for at least 1 week. In all our experiments, we used as control littermates mice carrying either no transgene, or the tTA or tetO transgene alone. Behavioural testing and the ChIP-seq experiment were performed with males. In all other experiments, mice from both sexes were used, keeping a balance between control and mutant groups. Mice were at least 2–4 months old unless indicated otherwise, except for the electrophysiological recordings conducted in younger animals (4–5 weeks old). Experimenters were blind to genotypes and the result of the PCR-based genotyping (see Supplementary Table 4 for primers sequences) was provided as a factor for statistical analysis once the experiments were concluded. Sodium butyrate (1.2 g kg −1 ) and buspirone (2 mg kg −1 ) were dissolved in PBS and administered by intraperitoneal injection. Mice were maintained according to animal care standards established by the European Union; all experimental protocols were approved by the Institutional Animal Care and Use Committee. Neuronal and cell line cultures Primary hippocampal neurons from Swiss albino mouse embryos at E17.5–E18.5 were cultured in 24-well plates (Becton Dickinson 353047) on 12 mm glass coverslips (VWR) coated with poly- D -lysine (Sigma Aldrich). After tissue homogenization, cells were counted in a Neubauer chamber and seeded at a density of ~130,000 cells per well. After 2–3 h, plating medium (DMEM supplemented with 10% fetal bovine serum, 0.45% glucose, 2 mM glutamine and penicillin/streptomycin 100 U ml −1 –100 μg ml −1 ) was replaced with defined maintenance medium (neurobasal supplemented with B27, 2 mM glutamine and penicillin/streptomycin 100 U ml −1 –100 μg ml −1 ). Transient transfection experiments in HEK293 cells, Neuro 2A (N2A) cells and primary hippocampal neurons with the plasmid pCAG-hH2BGFP were performed using Lipofectamine 2000 (Invitrogen). For N2A differentiation experiments, cells were transiently transfected with pCAG-hH2BGFP and planted on glass slides (1 × 10 4 cells per ml) in DMEM+1% fetal bovine serum; dibutyryl-cAMP (2.5 mM, Sigma) was added to the medium to stop proliferation and trigger differentiation towards a neuronal phenotype. Samples were fixed at indicated time points with 4% paraformaldehyde (PFA) and stained with Phalloidin-TRITC (10 μg ml −1 , Sigma) and DAPI (1 nM, Invitrogen) to visualize cell actin and DNA, respectively. RT–qPCR and ChIP–qPCR assays Extraction of hippocampal RNA and RT–qPCR assays were performed as previously described [49] . Primer sequences are listed in Supplementary Table 4 . For ChIP assays, mice were killed by decapitation and the whole hippocampus was dissected, minced into small pieces and cross-linked in 1% formaldehyde for 15 min at room temperature (at least three independent tissue samples per condition). Chromatin samples were then sonicated with a bioruptor (Diagenode) and incubated overnight at 4 °C in the presence of specific antibodies ( Supplementary Table 5 ) or rabbit-derived pre-immune serum. ChIP–qPCR assays were performed using specific primers immediately upstream of the transcription start site ( Supplementary Table 4 ). Microarray, ChIP-seq and other genomic analyses For microarray hybridization, total hippocampal RNA was extracted with TRI reagent (Sigma). Equal amounts of purified total RNA from a couple (one male and one female) of age and genotype-matched mice were pooled, treated with DNaseI and cleaned up using the RNeasy mini kit (Qiagen). Three independent pooled samples per genotype were hybridized to Mouse Gene 1.0 ST expression arrays (Affymetrix). Microarray data were analysed using the Bioconductor R packages oligo, genefilter and limma [50] . More precisely, expression data were preprocessed with Robust Multi-array Average (RMA) using the median polish method for probe-set summarization [51] ; then, control probes were removed and intensity filtering was applied to eliminate non-expressed probe sets (intensity value below 20% percentile in all arrays); finally, differential expression analysis was performed with moderated t -statistics [52] . Adjusted P -values were used to rank and filter expression values. Functional genomics enrichment analyses were performed at WebGestalt ( http://bioinfo.vanderbilt.edu/webgestalt/ ) [53] . ChIP-seq analysis was performed as in ref. 27 . Briefly, we pooled hippocampal chromatin of 12 male mice per condition. The cross-linked and sonicated chromatin was immunoprecipitated using a ChIP-grade (ChIP-seq tested) antibody against H3K27me3 (Abcam, ab6002, 1:100 dilution) or rabbit-derived preimmune serum. DNA libraries were produced and sequenced using a HiSeq-2500 apparatus (Illumina, service provided by Fasteris S.L.) according to manufacturer’s instructions. Two independent sequencing runs (1 × 50 bp) were performed for each library (technical replicates). Reads were mapped onto the mouse genome (NCBIM37/mm9) using BWA [54] , BAM files were generated and parsed to filter uniquely mapped reads using SAMTOOLS [55] and the heatmaps and k-means clustering analysis were performed on the merged replicates (library size >25 × 10 6 in all cases) using seqMINER [56] . Clusters showing H3K27me3 enrichment were merged for further analysis. Density plots showing intergenic distance were generated using the Refseq database after removal of overlapping genes. To evaluate a selective enrichment in genes with a long-distance neighbour among the differentially expressed genes in H2BGFP mice, we performed Fisher’s exact test against those genes contained in the array. The information about lamina-associated domains (LADs) was extracted from ref. 57 , about cis -regulatory elements from ref. 28 and the enrichment profiles for H3K9,14ac and H3K4me3 from ref. 27 . Microarray and ChIP-seq data is accessible through the Gene Expression Omnibus database using the accession number GSE56810. Molecular modelling For GFP docking into the nucleosome model, a homology model of GFP plus the 8-residue linker was built with MODELLER [58] using as template Protein Data Bank entry 4en1 with a sequence identity of 95%. Next, the modelled GFP domain was docked to the carboxy terminus of H2B (chain D of PDB entry 1ZBB) with pyDockTET [59] . Nucleosome radius increments were estimated by measuring interatomic distances, while volumes were calculated with help from UnionBalls [60] . FISH and immuno-FISH The FISH procedure was performed in 40 μm coronal brain cryosections of 4% PFA-perfused animals. The pancentromeric probe (Chrombios), directly labelled with Texas Red and recognizing a conserved sequence in mouse centromeres, was used according to manufacturer’s instructions. The CH29-584 BAC used as template for Htr1a probe was obtained from the Children’s Hospital Oakland Research Institute. For DNA amplification, Illustra Genomi Phi V2 kit (GE Healthcare) was used according to manufacturer’s protocol. The probe was directly labelled with Cy5-dUTP nucleotide using the Nick-Translation Mix (Roche). Htr1a-Cy5-labelled probe was verified on mouse metaphase spreads. The hybridization reaction was performed for 72 h with the probe diluted in buffer containing 50% formamide, 10% dextran and 2 × SSC (Sigma), followed by a series of high-stringency washes with 2 × SSC at 37 °C and 0.1 × SSC at 60 °C [61] . In immuno-FISH experiments, FISH was followed by a rabbit polyclonal antibody directed against the phosphorylated RNA pol II C-terminal domain phosphorylated on S2, or phosphorylated on S5, (Abcam), followed by DyLight 488-conjugated goat anti-rabbit antibody (Invitrogen), according to our standard protocol [62] . Nuclei were counterstained using Hoechst 33342 (Invitrogen). The quantitative analyses were performed using the public domain software Fiji ( http://fiji.sc/Fiji ) in 72 nuclei from control animals and in 86 nuclei from H2BGFP animals. Co-localization maps were made using the Fiji plugin parison with control group unless indicated otherwise. Other immunological methods Hippocampal protein extracts and western blot analysis were performed according to standard protocols. We used the primary antibodies listed in Supplementary Table 5 and horseradish peroxidase-conjugated secondary antibodies from Sigma-Aldrich. Flow cytometry experiments were performed in a BD FACSAria III apparatus and analysed using FACSDiva software. The initial steps of nuclei preparation for flow cytometry analysis were the same than in the ChIP procedure. To extract chromatin proteins and allow full access of PI (Sigma, P4170) to DNA, fixed nuclei were pre-incubated with 0.1 N HCl for 1 min (ref. 63 ). For immunohistochemistry, mice were anaesthetized with a ketamine/xylazine mixture and perfused with PFA (4% in 0.1 M phosphate buffer (PB)); brains were postfixed overnight and cut in a vibratome. Brain slices were washed with PBS, permeabilized with PBS containing 0.25% Triton X-100, incubated with the primary antibodies listed in Supplementary Table 5 and counterstained with a 1-nM DAPI (Invitrogen). For image acquisition, fluorescent specimens were examined under Carl Zeiss LSM780 Spectral Confocal using diode laser 405 nm (CW/pulsed), Diode-pumped solid-state 561 nm and HeNe 633 nm laser, at room temperature. Cross-talk between the fluorophores was avoided by adjustment of the spectral ranges of the detectors and sequential scanning of the images. Signal intensity quantification in individual nuclei (at least 20–30 nuclei per condition) was performed using the free open source application ImageJ64 as described [61] . Image stacks were acquired at the sampling density of 80 nm per pixel and Z -spacing of 200 nm, using Plan Apochromat × 63/1.4 Oil differential interference contrast (DIC) objective. To reduce noise and improve resolution, the stacks were 3D deconvolved by means of Huygens Professional software (Scientific Volume Imaging). Three-dimensional image analysis was performed in 221 nuclei from control animals and in 284 nuclei from H2BGFP animals using the custom-written software ‘Segmentation magick’ essentially as described in ref. 19 , except that the nucleus boundary had to be enhanced using anti-lamin B immunostaining because of the aberrant chromatin pattern in H2BGFP mice. The 3D reconstructions and movies were made using Imaris software (Bitplane). Other histological techniques For Nissl staining, brain slices were incubated with cresylviolet for 30 min, then dipped briefly in dH2O, washed briefly in 0.1% acetate in 95% ethanol, washed in 95% ethanol, washed in 100% ethanol, dipped in xylene twice for 3 min and quick mounted with Neo-Mount. For EM, bitransgenic and control littermates were perfused with 4% PFA and 1% glutaraldehyde in 0.1 M PB. Coronal sections were cut with a thickness of 60 μm at the level of the dorsal hippocampus. After several washes in PB, the sections were postfixed with osmium tetraoxide (1% in PB) and block stained with uranyl acetate (1% in distilled water). The sections were then dehydrated in ascending series of ethanol to 100% followed by propylene oxide, and flat embedded on glass slides in Durcupan. The CA1 region of the hippocampus was cut at 70–90 nm on an ultramicrotome and collected on 200-mesh nickel grids. Staining was performed on drops of 1% aqueous uranyl acetate followed by Reynolds’s lead citrate. Ultrastructural analyses were performed with a Jeol-1010 electron microscope. Electrophysiology Cortical slices of 300 μm thickness were prepared from H2BGFP and control littermates aged 4–5 weeks according to routine methods used in our laboratory [62] . Animals were killed by cervical dislocation, and coronal slices in which the hippocampus was present were cut with a Vibratome (Leica VT1000) in ice-cold cutting solution (composition in mM: NaCl, 124; KCl, 2.5; PO 4 H 2 Na, 1.25; MgCl 2 , 2.5; CaCl 2 , 0.5; NaCO 3 H, 26; glucose, 10; pH 7.4 when saturated with 95% O 2 and 5% CO 2 ). The slices were transferred to artificial cerebrospinal fluid (ACSF composition in mM: NaCl, 124; KCl 2.5; PO 4 H 2 Na, 1.25; Mg Cl 2 , 1; CaCl 2 , 2; NaCO 3 H, 26; glucose, 10; pH 7.4 when saturated with 95% O 2 and 5% CO 2 ) where they were incubated at 37 °C during 30 min and thereafter kept at room temperature until use. For recording, the slices were placed in a submersion type chamber, placed on the stage of an upright microscope (Olympus BX50WI) and superfused at a flow rate of 3–5 ml min −1 with ACSF at 33–34 °C. Hippocampal CA1 pyramidal neurons were identified visually with DIC optics and infrared illumination. Intracellular recordings were obtained with glass microelectrodes pulled in a Sutter P-97 electronic puller (Sutter Instruments, USA) that had a resistance of 3–7 MOhm when filled with intracellular solution (Composition in mM: KMeSO 4 , 135; NaCl, 8; HEPES, 10; Mg 2 ATP, 2; Na 3 GTP, 0.3; pH 7.3 adjusted with KOH; osmolality 295 mOsm kg −1 ). Current clamp recordings were acquired with a two channel Multiclamp 700B amplifier (Axon Instruments, Molecular Devices, USA), low pass filtered at 6 KHz and digitized at 20 KHz with a Digidata 1322A (Axon Instruments, Molecular Devices). Serotonin was obtained from Sigma-Aldrich (USA) and applied dissolved in ACSF at a final concentration of 5 μM. Each slice was used only for the recording of a single neuron to avoid possible long-term effects of the serotonin on the electrophysiological properties of CA1 pyramidal neurons. Membrane input resistance was measured using hyperpolarizing current pulses of 25 pA and 250 ms. In some recordings, during the serotonin application the membrane potential was adjusted to the resting level with direct current injection. Statistical comparisons were made with SigmaStat 3.2 (Systat Software Inc.); Student’s t -test for unpaired and paired samples were used after checking for the normality and equal variance of the samples; data are given as mean±s.e.m. Behavioural analysis Three independent cohorts of adult (3–6 months old) bitransgenic and control littermate males were tested in series of behavioural tasks. Cohort 1: Open field (OF), Elevated Plus Maze, Rotarod, SHIRPA, Forced Swim Test, Tail Suspension Test and Hot Plate Test; Cohort 2: Morris Water Maze (including visible and hidden platform tasks), Stress-induced Hyperthermia (SIH), Social Interaction, Marble Burying and Novel Object Exploration tests; Cohort 3: Startle Response and Prepulse Inhibition, NOR memory test, Three-chambered Social Approach test and Fear Conditioning (including contextual and cued tests). Mice from the three cohorts were finally used in experiment evaluating the interaction of the 5-HT1A receptor agonist buspirone with relevant behaviours. Buspirone (2 mg kg −1 ) was administered 20 min before a new 30-min OF session to examine the impact in locomotor hyperactivity. Immediately after, one 3-week-old mouse was brought in the centre of the chamber to evaluate social interaction. The SHIRPA primary screen, OF, Elevated Plus Maze and Fear conditioning tasks were performed as previously described [64] . To study motor coordination and learning, mice were trained on a Rotarod (Ugo Basile) at a constant speed (4 r.p.m.) four times per day during 2 days. On the testing day, the Rotarod was set to increase its speed 1 r.p.m. every 16 s starting at 4 r.p.m., and the latency to fall was measured. To evaluate nociception and sensitivity to thermal stimulus, mice were placed in the test chamber of a hot plate (IITC Life Science) set at 54 °C, and the latency until the animal exhibited paw licking was recorded. All mice were tested three times with 1 h interval between each measurement. Spatial learning in the Morris Water Maze was assessed in a circular tank (170 cm diameter) filled with opaque white water as described previously [64] . Mice were monitored throughout the training and testing sessions with the video-tracking software SMART (Panlab S.L.). A platform of 10 cm diameter was submerged 1 cm below the water surface in the centre of the target quadrant. The training protocol, both when the platform was visible (5 d: V1 to V5) and hidden (8 d: H1 to H8), consisted of four trials per day with a 45-min intertrial interval. If the mice did not find the platform after 120 s, they were gently guided to it. Mice were transferred to their cages only after remaining on the platform for at least 10 s. Memory retention trials of 60 s were performed at the beginning of day H5 (probe trial 1) and 24 h after concluding the training on day H8 (probe trial 2). The NOR task was performed as previously described [65] with a 10-min training session and a 10-min testing session 24 h after training. For Forced Swim Test, mice were placed into clear plastic buckets 2/3 filled with 26 °C water and videotaped from the side. After 2 min pretest period, the activity of the mice the following 4 min was scored. Tail Suspension Test was performed with Med associates Inc. equipment; mice were suspended by the tail with adhesive tape to a hook connected to a strain gauge during 6 min and their activity recorded. To evaluate physiological mild stress, SIH was evaluated by measuring rectal temperature twice with an intertrial interval of 10 min in which the mice were placed in a new cage; the difference (Δ T = T 2− T 1) reflects the SIH response. In both the social interaction test and novel object tests, mice were placed in a white acrylic box (48 × 48 × 30 cm) for 30 min of habituation; then, either a 3-week-old mouse or a novel object was introduced in the cage and the number of contacts and the latency until the first investigation were measured. In the marble-burying task, 16 opaque marbles were placed in a 4 × 4 arrangement (5 cm separation between marbles) on top of fresh sawdust; then, the number of marbles with more than 2/3 of their surface covered with sawdust (buried) during the 30-min test session was scored. Prepulse inhibition was carried as previously described [64] but using different intensity for the prepulse: 20-ms prepulse trials of 83, 86 and 92 dB. In the three-chambered social approach test, mice were initially placed in the centre chamber with access to two side chambers containing one empty cylinder; after 5 min of freely exploring this environment (Hab), an unfamiliar C57BL/6J male mouse (Mouse1) was placed in one of the empty cylinders for 10 min and the time spent interacting with the empty or the occupied cylinder was scored (Test1). Immediately after, a second unfamiliar male (Mouse2) was placed inside the empty cylinder to evaluate social novelty during 10 min; the time spent interacting with stranger 1 and 2 was scored (Test2). Accession codes: Microarray and ChIP-seq data is accessible through the Gene Expression Omnibus (GEO) database using the accession number GSE56810 . How to cite this article: Ito, S. et al. Loss of neuronal 3D chromatin organization causes transcriptional and behavioural deficits related to serotonergic dysfunction. Nat. Commun. 5:4450 doi: 10.1038/ncomms5450 (2014).